RETRACTED ARTICLE: REST regulates the cell cycle for cardiac development and regeneration Despite the importance of cardiomyocyte proliferation in cardiac development and regeneration, the mechanisms that promote cardiomyocyte cell cycle remain incompletely understood. RE1 silencing transcription factor (REST) is a transcriptional repressor of neuronal genes. Here we show that REST also regulates the cardiomyocyte cell cycle. REST binds and represses the cell cycle inhibitor gene p21 and is required for mouse cardiac development and regeneration. Rest deletion de-represses p21 and inhibits the cardiomyocyte cell cycle and proliferation in embryonic or regenerating hearts. By contrast, REST overexpression in cultured cardiomyocytes represses p21 and increases proliferation. We further show that p21 knockout rescues cardiomyocyte cell cycle and proliferation defects resulting from Rest deletion. Our study reveals a REST-p21 regulatory axis as a mechanism for cell cycle progression in cardiomyocytes, which might be exploited therapeutically to enhance cardiac regeneration. Cardiomyocyte proliferation is required for generating myocardial mass and building a functional four-chamber heart during embryonic development [1] , [2] , [3] . After birth, cardiomyocytes continue to proliferate in a short neonatal period, which is crucial for the final cardiac growth surge as well as for regeneration of injured mouse neonatal hearts [4] , [5] , [6] . The vast majority of cardiomyocytes then exits the cell cycle and stops proliferating after preadolescence [7] , [8] , [9] , [10] . The inability of cardiomyocytes to proliferate prevents the replenishment of lost or dysfunctional cells in a diseased heart [11] . Because heart diseases are the number one cause of death worldwide [11] , it is important to identify the regulatory factors of the cardiomyocyte cell cycle, which may be used as therapeutic targets for these devastating conditions. Several transcription factors, such as GATA4 [12] , TBX20 [13] , BRG1 [14] , YAP [15] , [16] , ERBB2 [17] , PITX2 [18] , and MEIS1 [19] have been shown to be essential for cardiomyocyte proliferation during development and for regeneration following neonatal heart injury. Transcriptional repressor element-1 silencing transcription factor (REST), also known as neuron-restrictive silencer factor (NRSF), is widely expressed in the embryonic tissues [20] , [21] . It binds a cis -element of 21 nucleotide base pairs, named RE1 motif [22] , to silence the expression of neuronal genes in the non-neuronal cells required for neurogenesis [23] , [24] . We have recently reported REST acting as a transcription repressor in mouse embryonic hearts [20] . In this study, we reveal that suppression of the cell cycle inhibitor gene p21 by REST is critically required during cardiac development and regeneration to maintain cardiomyocyte proliferation. We show that REST binds and represses the cell cycle inhibitor gene p21 , which is required for mouse cardiac development and regeneration. Rest deletion de-represses p21 and inhibits the cardiomyocyte cell cycle and proliferation in embryonic or regenerating mouse hearts. We also show that p21 knockout rescues the cardiomyocyte cell cycle and proliferation defects resulting from Rest deletion. By elucidating the REST-p21 genetic mechanism underlying the cell cycle regulation of proliferating cardiomyocytes during cardiac development and regeneration, our study provides an opportunity for developing cell-based therapeutics for heart disease. Rest is required for embryonic cardiomyocyte proliferation Our recent studies showed that REST represses transcription in mouse embryonic hearts [20] . Based upon this, we did a time course of REST expression levels at various developmental stages. By western blot, we found that REST was downregulated in the ventricles of neonatal hearts (Supplementary Fig. 1a, b ). Further, immunostaining showed that REST was expressed in the majority of cardiomyocytes between embryonic day (E) 11.5 and postnatal day (P) 3, whereas the number of REST-expressing cardiomyocytes was drastically reduced from P3 to P28 (Supplementary Fig. 1c, d ). The downregulation of REST protein level was not accompanied by a change in mRNA level (Supplementary Fig. 1e ), and was possibly due to the REST protein degradation [21] , [25] . Given that downregulation of REST coincided with the cell cycle exit of cardiomyocytes [5] , we examined the relationship of REST expression with cardiomyocyte proliferation by immunostaining. The results revealed that the majority of EdU+ proliferating cells expressed REST (Supplementary Fig. 2a–c ). We next inactivated Rest in the myocardium ( Rest mKO ) using TnT Cre and Rest GT/GT mice [23] to determine its role in cardiomyocytes and confirmed that Rest was effectively deleted in the myocardium by immunostaining and western blot (Fig. 1a, b ). Rest mKO embryos were runted and >80% of them were dead by E16.5 (Fig. 1c ). Rest mKO hearts at E10.5–12.5 had thin ventricular walls and defective trabeculae (Fig. 1d, e ). Notably, there was significantly reduced percentage of Rest mKO cardiomyocytes that were expressing the cell cycle markers (Ki67 for cell cycle activity, EdU for DNA synthesis, pH3 for mitosis, and Aurora B for cytokinesis) (Fig. 1f ). Such proliferation defect was not associated with changes in myocardial differentiation and apoptosis (Supplementary Fig. 3a–g ). These observations demonstrate that Rest is essential for embryonic cardiomyocyte proliferation and chamber development. Fig. 1 Rest is required for myocardial development and cardiomyocyte proliferation. a , b Immunostaining and western blot analyses showing the efficient deletion of Rest in cardiomyocytes in TnT Cre ; Rest GT/GT ( Rest mKO ) hearts. Controls were Rest GT/GT mice. c A summarizing graph of the distribution and number of embryos at different stages indicates death of Rest mko embryos between E12.5 and E16.5. d , e H&E-stained sections of E10.5 and E12.5 hearts indicate thin ventricular wall resulting from Rest deletion. f Quantitative immunostaining of cell cycle markers showing reduced proliferation of Rest mKO cardiomyocytes. n = 4/group, mean ± s.d., * p < 0.05 by unpaired two-tailed Student’s t test. Scale bars = 40 µm Full size image Rest is required for neonatal cardiomyocyte proliferation To determine whether Rest is also requirement for neonatal cardiomyocyte proliferation, we deleted Rest at P1, P3, or P7 using an inducible TnT MerCreMer driver ( Rest imKO , thereafter) (Fig. 2a, b ). Rest inactivation at P1, but not at P3 or P7, resulted in the death of ~80% of neonates within 1 week after tamoxifen injection (Fig. 2c ). Based upon this, we focused on inactivating Rest at P1 and investigating the resultant changes in cardiac morphology and function at P3. H&E staining showed that the Rest imKO hearts were underdeveloped with a reduced ratio of the heart/body weight (Fig. 2d ). Echocardiography revealed a noticeable reduction in the left ventricular mass, left ventricular wall thickness, and contractility (Fig. 2e–g ). Flow cytometry assays further revealed a reduced percentage of cardiomyocytes in Rest imKO hearts (Fig. 2h ). The null cardiomyocytes were accumulated at the G0/G1 phase of cell cycle, while their presence at the S and G2/M phases was reduced (Fig. 2i, j ). Immunostaining for Ki67 and EdU confirmed the cell cycle defect (Fig. 2k ). In contrast, Rest deletion at P3 or P7, when cardiomyocytes were exiting the cell cycle, had no effect on cardiac morphology and function (Supplementary Fig. 4a–d ). Therefore, Rest is also required for neonatal cardiomyocyte proliferation through maintaining cell cycle progression, and neonatal cardiac growth and function. Fig. 2 Rest is required for neonatal cardiomyocyte proliferation and cardiac function. a A graph of experimental design for generating myocardial Rest knockout ( Rest imKO ) at different postnatal (P) stages using the inducible TnT MerCreMer deleter mice. b Western blots showing effective deletion of Rest . c Survival curve of control and Rest imKO mice, p < 0.001, log-rank (Mantel–Cox) testing between mice with Rest deletion at different stages and control (Tam-treated Rest +/+ ;TnT MerCreMer /+ mice). d Representative H&E staining and heart/body weight ratio revealing underdeveloped Rest imKO hearts at P3 after Rest deletion at P1. n = 5/group. Scale bar = 100 µm. e – g Echocardiography showing structure defects and decreased left ventricle function of P3 Rest imKO . n = 6 for Rest imKO ; n = 8 for Control. h – j FACS shows reduced percentage of cardiomyocytes isolated from P3 Rest imKO hearts ( h ) and arrested cell cycle of the Rest imKO cardiomyocytes at G0/G1 phase ( i , j ). k Immunostaining for cell cycle markers indicating reduced proliferation of Rest null cardiomyocytes. n = 4/group for FACS and immunostaining. Scale bar = 40 µm. Mean ± s.d., * p < 0.05, unpaired two-tailed Student’s t test Full size image REST binds and represses p21 to regulate cardiomyocyte proliferation To identify the downstream factor(s) of REST involved in the cell cycle regulation, we re-analyzed our previously published RNA-seq data from E12.5 control versus Rest mKO hearts [20] and found that p21 ( Cdkn1a ) was the only cell cycle inhibitor gene significantly upregulated in Rest null hearts, whereas the expression of several cell cycle activators was downregulated (Supplementary Fig. 5a ). These findings were then confirmed by qRT-PCR (Supplementary Fig. 5b, c ). Notably, p21 was also the only cell cycle inhibitor gene which expression was significantly upregulated in P2 ventricles with myocardial Rest inactivation at P1 (Supplementary Fig. 5d ). Immunostaining further showed an increased number of p21 -expressing cardiomyocytes in E12.5 and P3 Rest null hearts (Fig. 3a, b ). We identified one conserved REST-binding site (RE1 motif) located at the 3′ end of mouse p21 gene by sequence alignment between mouse and human (Fig. 3c ). Luciferase reporter gene assays and mutational analyses revealed that the p21 -RE1 motif was required for repressing transcription in cultured P1 mouse cardiomyocytes (Fig. 3d ). Quantitative chromatin immunoprecipitation assays (qChIP) showed REST occupancy of the p21 -RE1 motif in E12.5 and P1 ventricles, but the occupancy was greatly reduced in the ventricles of P21 when REST level was largely diminished (Fig. 3e ). Further, qChIP showed that Rest deletion resulted in an enrichment of H3K4me3 histone modification and a reduction of H3K9me3 and H3K27me3 histone marks at the p21-RE1 motif (Fig. 3f ). These findings support that REST directly binds p21 and represses its transcription in cardiomyocytes, possibly through histone methylation changes [26] . Fig. 3 REST binds p21 to repress its expression. a , b Immunostaining ( n = 4/group) showing upregulated p21 protein level in the Rest deleted E12.5 and P3 hearts. Scale bar = 40 µm. c Top, Sequence alignment of p21 between mouse and human indicating a conserved RE-1 motif (red vertical line) located at the 3′ UTR. Bottom, The p21- RE1 motif and its mutated (Mut) or deleted (Del) counterpart. d Luciferase reporter assays with a 690-bp mouse DNA fragment containing the wild type (WT), mutated, or deleted RE1 motif reveals that the intact p21- RE1 motif is required for repressing the reporter gene transcription in primary cultured P1 mouse cardiomyocytes. e qChIP using REST antibodies indicates enrichment of p21- RE1 motif containing DNA fragments in the ventricles of E12.5 and P1, but not P21. f qChIP with P2 ventricles using the REST and histone mark antibodies showing the REST-dependent histone modification of the p21- RE1 motif. n = 3/group for d – f , mean ± s.d., * p < 0.05 by one-way ANOVA followed by Tukey’s test in d ; unpaired Student’s t test in b , e , f . NS no significance Full size image To determine whether such repression promoted cardiomyocyte proliferation during cardiac development, we deleted p21 in Rest mKO mice by breeding them with p21 knockout mice [27] . Inactivation of p21 rescued embryonic lethality and cardiac phenotypes of Rest mKO mice at E12.5 (Fig. 4a–c ). Inactivation of p21 also restored the levels of Cyclin B, Cyclin E, and CDK1/2 (Fig. 4d ), and re-established normal cardiomyocyte cell cycle and proliferation, as indicated by recovered expression of Ki67, PH3, and Aurora B, and EdU incorporation (Fig. 4e ). Double knockout (DKO) mice were survived to birth and appeared healthy postnatally and in adulthood, with normal cardiac morphology, heart/body weight ratio, and cardiac function (Fig. 4f–i ). Similarly, inactivation of p21 rescued postnatal lethality of mice caused by inactivation of myocardial Rest at P1 (Fig. 5a ). Cardiac phenotypes were rescued, including the cardiac size, heart/body ratio, cardiac function (Fig. 5b–e ), as well as the expression of cell cycle activators and markers (Fig. 5f, g ). We also examined whether forced overexpression of REST would promote cardiomyocyte proliferation in cultured cardiomyocytes isolated from P1 or P5 hearts. We first treated the culture with siRNAs against β-TrCP that mediates REST degradation via ubiquitination [21] , [25] . The results of western blot for REST, qRT-PCR for Rest , and REST-targeted genes and immunostaining for EdU and PH3 showed that downregulation of β-TrCP slowed down the REST degradation (Supplementary Fig. 6a ), suppressed the expression of REST target genes ( Hcn2, p21, Nppa , and Syn1 ) (Supplementary Fig. 6b ), and upregulated cardiomyocyte proliferation (Supplementary Fig. 6c ). Next, we overexpressed REST by transfection of a plasmid (pHR-NRSF-CITE-GFP) containing Rest cDNA [28] and found by western blot and immunostaining for EdU and PH3 that overexpression of REST dose-dependently repressed p21 expression and increased cardiomyocyte proliferation (Supplementary Fig. 6d–f ). These findings, therefore, identify that a Rest-p21 axis underlies the regulation of cardiomyocyte cell cycle for fetal and neonatal cardiac development. Fig. 4 p21 deletion rescues embryonic heart defects resulting from myocardial Rest deletion. a Survival curve, no difference between control and p21 null ( p21 KO ) or p21/Rest double knockout ( DKO ) group by log-rank (Mantel–Cox) test. p < 0.001 between Rest mKO and each of other groups. b , c H&E-stained E12.5 heart sections showing that thin ventricular walls of Rest deleted hearts are restored by p21 deletion ( n = 3/group). Scale bar = 100 μm. d Representative western blot revealing that upregulation of p21 and downregulation of Cyclin B, Cyclin E, and CDK1/2 in E12.5 Rest null hearts are restored to the normal levels of control hearts by p21 deletion. e Immunostaining for cell cycle markers indicating that p21 inactivation rescues the cell cycle defect resulting from Rest deletion ( n = 4/group). Scale bar = 40 μm. f – i H&E staining ( f scale bar = 100 μm), ratio of heart/body weight ( g ), and echocardiography ( h , i ) showing that P28 Rest / p21 DKO mice have cardiac structure and function comparable to control littermates ( n = 6–8/group). Mean ± s.d. * p < 0.05 by one-way ANOVA followed by Tukey’s test. NS no significance Full size image Fig. 5 p21 deletion rescues neonatal heart defects resulting from Rest deletion. a Survival curve, no difference between control and p21 null ( p21 KO ) or p21/Rest double knockout ( DKO ) group by log-rank (Mantel–Cox) test. p < 0.001 between Rest imKO and each of other groups. b , c H&E-stained P3 heart sections showing that underdeveloped Rest null hearts are restored by p21 deletion ( n = 5/group). Scale bar = 100 μm. d , e Echocardiograph showing p21 knockout rescues cardiac function resulting from Rest deletion at P1 ( n = 6–8/group). f Representative western blot revealing upregulation of p21 and downregulation of Cyclin B, Cyclin E, and CDK1/2 in P3 Rest null hearts are restored by p21 deletion to the normal levels of control hearts. g Immunostaining for cell cycle markers indicating p21 inactivation rescues the cell cycle defect resulting from Rest deletion ( n = 4/group). Scale bar = 40 μm. Controls were the Tam-treated Rest +/+ ; TnT MerCreMer/+ mice. Mean ± s.d. * p < 0.05 by one-way ANOVA followed by Tukey’s test Full size image Rest is required for regenerative cardiomyocyte proliferation To further investigate whether REST had a role in cardiac regeneration, we investigated Rest expression in repairing neonatal hearts using an apical resection model [4] . Consistent with previous reports [4] , [6] , immunostaining for the cell cycle markers showed a significantly increased number of cardiomyocytes that re-entered the cell cycle in the injured region at P7, 3 days after ablation at P4 (Fig. 6a ). Notably, the number of REST-expressing cardiomyocytes was also increased in the same region and was correlated with the increased number of cells undergoing DNA synthesis, mitosis, and division (Fig. 6b ). The percentage of EdU+ cells that also expressed REST was sustained in the regenerating myocardium from P7 to P28 (Fig. 6c ). About 90% of REST-expressing cells in the apex undergoing repair were cardiomyocytes; the reminder was epicardial or endocardial cells (Supplementary Fig. 7a–d ). These findings indicated that the majority of REST-expressing cells were proliferating cardiomyocytes induced by injury. We deleted Rest in the myocardium at P3 and performed apical resection at P4. The P3 deletion bypassed the death of neonates when Rest was deleted at P1, while apical ablation at P4 was still within the window of myocardial regeneration [2] . We found by Masson’s trichrome staining that the fibrotic scar in the apex of Rest null hearts ( Rest imKO ) was not resolved at P14 and P28 compared to the control hearts (Fig. 7a, b ). Consistent with the persistent scaring phenotype, Rest imKO hearts had reduced left ventricular function as observed by echocardiography (Fig. 7c, d ). Further, immunostaining revealed that the number of EdU+ proliferating cardiomyocytes in the injured apex of Rest imKO hearts was significantly reduced (Fig. 7e–g ). Together, these findings suggest that REST re-expression is necessary for the regeneration of neonatal hearts. Fig. 6 Co-upregulation of REST and cardiomyocyte proliferation in injured neonatal hearts. a , b Quantitative immunofluorescence ( a Scale bar = 40 μm.) and scatter plot b showing increased expression of REST and its positive relation with the expression of cell cycle markers in cardiomyocytes. Average counts from six fields/section, four sections/ventricle, four ventricles/stage at P7, P14, and P28, mean ± s.d. * p < 0.05 by one-way ANOVA followed by Tukey’s test. APB/APR apex border/apex remote. c Co-immunofluorescence showing consistently ~60% of EdU+ cells express REST (arrow) in regenerating neonatal hearts. Scale bar = 10 μm. Data are presented as mean ± s.d. ( n = 4/stage) Full size image Fig. 7 Rest is required for regeneration of injured neonatal hearts. a , b Quantitative Masson’s trichrome staining shows increased cardiac fibrosis in mice with induced myocardial Rest deletion at P3 and injured by apex ablation at P4, n = 5–8/group. Scale bar = 100 μm. c , d Echocardiography indicating reduced cardiac function of myocardial Rest null mice after injury, n = 6–8/group. e – g Quantitative immunofluorescence ( n = 4/group) showing decreased EdU+ cardiomyocytes in regenerating hearts in mice with Rest deletion. Scale bar = 40 μm. Mean ± s.d. p < 0.05 by two-way ANOVA followed by Sidak’s test in b – d ; unpaired two-tailed Student’s t test in f , g Full size image The increased number of REST-expressing cardiomyocytes in the regenerating neonatal hearts was correlated with increased REST occupancy at the p21- RE1 motif (Supplementary Fig. 8a ). Concurrently, the regenerating myocardium expressed a low level of p21 mRNA (Supplementary Fig. 8b ). Immunostaining also showed that the number of p21-expressing cardiomyocytes was negatively correlated with that of REST-expressing cells in the regenerating myocardium (Supplementary Fig. 8c, d ). In contrast, p21 transcription was de-repressed in the injured Rest imKO apex, which was accompanied with downregulation of the cell cycle activators (Supplementary Fig. 8e, f ). To determine whether p21 upregulation was responsible for the reduced proliferation of cardiomyocytes and poor regeneration of myocardium after Rest deletion, we performed the apical resection on the Rest and p21 DKO hearts at P4, 1 day after Rest deletion (Fig. 8a ). Like control hearts, p21 −/− hearts had normal left ventricular function at P28 (Fig. 8b, c ). We noted that p21 −/− hearts had less fibrotic scar tissue as compared to controls (Fig. 8d ). Importantly, p21 deletion improved regeneration and function of Rest imKO hearts and restored the number of EdU+ cardiomyocytes in the injured myocardium (Fig. 4e ). These results demonstrate that the Rest-p21 axis regulation of cardiomyocyte proliferation also underlies the neonatal cardiac regeneration. Fig. 8 REST-dependent p21 expression is required for cardiac regeneration. a Schematic diagram showing experimental procedure of cardiac apex resection (AR) on neonatal mice. b , c Echocardiography indicates that mice with control ( n = 9), single p21 knockout ( p21 KO , n = 8), and double knockout of Rest and p21 (DKO, n = 8) injured hearts have cardiac function comparable to that of the sham-operated control (s-Control, n = 9) at P28. Injured Rest single knockout ( Rest imKO , n = 9) hearts have significantly decreased left ventricular function comparable to injured control. d , e Quantitative Masson’s trichrome staining ( n = 8/group) ( d Scale bar = 100 µm) and EdU assays ( n = 4/group) ( e Scale bar = 40 µm) showing p21 inactivation reduces the cardiac fibrosis and rescues cardiomyocyte proliferation defect in the injured apex resulting from Rest deletion. Mean ± s.d. * p < 0.05 by one-way ANOVA followed by Bonferroni test. NS no significance Full size image Overall, our study identifies a molecular mechanism by which REST repression of the cell cycle inhibitor p21 is necessary and sufficient for promoting the cardiomyocyte cell cycle and proliferation during cardiac development and regeneration. p21 is a well known cell cycle inhibitor through interacting with the G1/M and G2/S CDK cyclins and inhibits their function to drive the cell cycle [29] . Of particular note, p21 is the only cell cycle inhibitor gene significantly repressed by REST in the proliferating cardiomyocytes during cardiac development and regeneration, suggesting that REST repression of p21 is a major mechanism underlying the regulation of cardiomyocyte cell cycle. Consistent with this notion, p21 deletion has been reported to enhance the regeneration of injured appendage [30] and neonatal hearts [31] . Interestingly, GATA4 [32] and MEIS1 [19] also repress p21 transcription in mouse embryonic and injured neonatal hearts, respectively. Since neither GATA4 nor MEIS1 expression is affected by REST inactivation, REST repression of p21 is likely independent of GATA4 and MEIS1. REST thus joins a network of transcription factors or cofactors, including MEIS1 [19] , YAP [15] , [16] , GATA4 [12] , [33] , [34] , and TBX20 [13] , as a new member essential for cardiac development and regeneration. Elucidating the Rest - p21 axis underlying the regulation of cardiomyocyte cell cycle may have clinical implications by providing an opportunity for better understanding of cardiomyocyte proliferation in cardiac regeneration. It is well known that the cell cycle arrest of cardiomyocytes is a normal physiological feature of adult hearts [5] . This, however, prevents the endogenous regeneration of infarcted adult hearts from the proliferation of pre-existing cardiomyocytes [11] , [35] . Our studies indicate that REST is rapidly diminished in the postnatal heart, but rebounded after injury. These observations suggest that REST downregulation might be one of the limiting factors for sustaining proliferation of postnatal cardiomyocytes. Future investigations are needed to determine whether REST is reactivated in adult hearts by injury and if the reactivation promotes adult cardiac regeneration by modulation of the activity of cardiomyocyte cell cycle. Mouse strains Floxed Rest mice ( Rest GT/GT ), which carries a conditional gene trap (GT) cassette [23] , were bred to TnT Cre [36] or TnT MerCreMer [37] mice to obtain Rest deletion in myocardium. Intraperitoneal tamoxifen (TAM) injection at 40 mg/kg was used for inducible inactivation. For rescue experiments, TnT Cre ; Rest GT/GT ( Rest mKO ), or TnT MerCreMer ;Rest GT/GT ( Rest i mKO ) mice were crossed to p21 −/− ( Cdkn1a − / − ) mice [27] . All mouse stains were in the C57B6 background. Embryos were isolated and inspected according to expected developmental ages. Age-matched embryos and neonatal mice of both sexes were grouped according to genotypes during experiments. Noontime on the day of detecting vaginal plugs was designated as E0.5, and morning on the day of observing newborns was designated as P0. 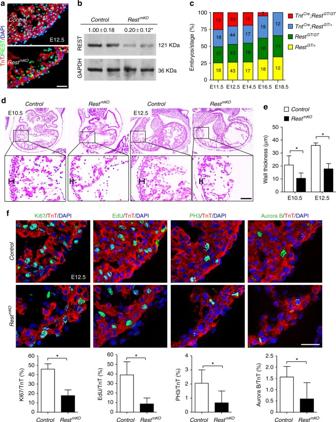Fig. 1 Restis required for myocardial development and cardiomyocyte proliferation.a,bImmunostaining and western blot analyses showing the efficient deletion ofRestin cardiomyocytes inTnTCre;RestGT/GT(RestmKO) hearts. Controls wereRestGT/GTmice.cA summarizing graph of the distribution and number of embryos at different stages indicates death ofRestmkoembryos between E12.5 and E16.5.d,eH&E-stained sections of E10.5 and E12.5 hearts indicate thin ventricular wall resulting fromRestdeletion.fQuantitative immunostaining of cell cycle markers showing reduced proliferation ofRestmKOcardiomyocytes.n= 4/group, mean ± s.d., *p< 0.05 by unpaired two-tailed Student’sttest. Scale bars = 40 µm The yolk sac or tail of mice was used for genotyping by PCR using Cre and allele-specific primers (Supplementary Table 1 ). Mouse housing and experiments were according to the protocols approved by the Institutional Animal Care and Use Committee (IACUC) of Albert Einstein College of Medicine. Neonatal heart apical resection Neonatal mouse heart apical resection (AR) was performed on postnatal day (P) 4 mice of both sexes as previously described [4] . Briefly, we induced deletion of Rest in the myocardium at P3 by tamoxifen and performed apical resection at P4. P4 neonates were anesthetized by inhalation of 2% isoflurane and 100% oxygen on ice and then subjected to intercostal incisions to separate the pericardium and expose the apex. The apex was amputated with microsurgical scissors under a dissecting microscope. About 10% of the heart was surgically removed to produce reproducible regeneration. The chest wall was then closed with sutures and the skin incision was closed using skin adhesive. After the operation, the neonates were placed back with the feeding female mice. Sham-operated mice underwent the same procedure without apical resection. Histology Embryos or isolated hearts were fixed in 4% paraformaldehyde (PFA), dehydration, embedded in paraffin, and sectioned frontally at 6-μm thickness. H&E and Masson’s trichrome staining were performed for detecting cardiac structure defects and fibrosis, respectively. The fibrotic area was quantified using the MetaMorph software (Molecular Devices). Primary cardiomyocyte cultures Cardiomyocytes (CMs) were isolated as described in previous studies [20] . Ventricles were dissected out from P1 or P5 neonates of both sexes, minced and dissociated by 0.045% collagenase II and 0.08% trypsin-EDTA at 37 °C. Non-CMs were removed through adhesive plating. Purified CMs were cultured in 12-well plates for 24 h at 37 °C with 5% CO 2 in Dulbecco’s modified Eagle’s minimum essential medium (DMEM) supplemented with 10% fetal calf serum. siRNA and cDNA transfection siRNA against β-TrCP ( si-β-TrCP , Santa Cruz Biotechnology) or plasmids containing mouse Rest cDNA (pHR-NRSF-CITE-GFP, Addgene) was transfected into cultured neonatal cardiomyocytes isolated from P1 or P5 neonatal hearts, at 70% confluency. Lipofectamine 3000 Regent (Invitrogen) and si-β-TrCP (40 nM) or REST-cDNA (0.5 or 2 µg/ml) were incubated in OPTIMEM (Invitrogen) for 15 min at RT, and then added to cells and incubated for indicated time. qRT-PCR and western blot were used to confirm the efficiency and effect of transfection. ChIP-qPCR ChIP-qPCR assays were performed as previously reported [38] . Ventricles (30–40 mg) from indicated stages were treated with 1% formaldehyde at room temperature for 10 min to crosslink protein and DNA complexes before quenched with addition of glycine. After three washes with PBS, tissues were homogenized, lysed, and sonicated to shear DNAs into 100–500 bp fragments. The DNA fragments were incubated with 5 µg antibodies against REST (EMD Millipore, 17–641, 1:100), Tri-Methyl-Histone H3 (Lys9) (CST mAb #13969, 1:100), Tri-Methyl-Histone H3 (Lys27) (CST mAb #9733, 1:100), Tri-Methyl-Histone H3 (Lys4) (CST mAb #9751, 1:100), or Acetyl-Histone H3 (Lys9) (CST mAb #9649, 1:100) overnight at 4 °C using Dynabead Protein G in a final volume of 500 µl and Magnet Starter Pack (Invitrogen, 10004D). Five microgram IgGs (Abcam, ab171870) were used as control. Immunoprecipitated DNAs were extracted and used for qPCR analysis to determine the enrichment of DNA fragments containing the p21-RE1 using specific primers (Supplementary Table 1 ). Western blot Ventricles were collected at the indicated stages, homogenized in radioimmunoprecipitation assay buffer at 4 °C and quantified by bicinchoninic acid assay. Equal total proteins (20 μg) were resolved in SDS-PAGE gels and transferred onto polyvinylidene fluoride membranes (Immobilon, Millipore). The membranes were blocked and incubated with primary antibodies at 4 °C overnight before incubated with HRP-conjugated secondary antibodies. Protein bands were detected by enhanced chemiluminescence. Antibodies, including REST (Antibodies-online, ABIN747683, 1:1000), P21 (Abcam, ab109199, 1:500), Cyclin E (Santa Cruz, sc-377100, 1:1000), Cyclin B (Santa Cruz, sc-166210, 1:1000), CDK1/CDK2 (Santa Cruz, sc-53219, 1:1000), and GAPDH (Thermo Fisher, MA5-15738, 1:5000), were used in western blot analysis. Full scans of western blots are shown in Supplementary Figs. 9 – 14 . Echocardiography Echocardiography was performed using a Vevo 770 ultrasound system (Visual Sonics, Toronto, Canada). Investigators were blinded to genotype and treatment groups. Mice were anesthetized with 1.5% isoflurane and mouse hearts were viewed on two-dimensional short-axis planes and measured using M-mode. Heart rate, left ventricular internal diameter, interventricular septal, and posterior wall (PW) dimensions were measured at end ystole and end diastole for at least three cardiac cycles. Fractional shortening (FS) were calculated by the average of FS measurements of the left ventricular contraction for five cardiac cycles. Quantitative reverse transcription PCR (qRT-PCR) Total RNAs were extracted from ventricles or cultured CMs using TRIzol (Life Technologies). One microgram of total RNAs was reverse transcribed to cDNA using a Superscript II reverse transcriptase Kit (Life Technologies). qRT-PCR was performed using Power SYBR Green PCR Master Mix (Life Technologies) and carried out on an Applied Biosystems 7900HT Fast Real-Time PCR System. Specific primers were listed in Supplementary Table 1 . The relative expression of each gene was normalized to the expression of Gapdh and calculated using the 2 − ΔΔCT method. Biological replicates were performed using three individual samples of each genotype and technical triplicates were carried out for each run of qPCR. Luciferase reporter gene assay Transcriptional suppression of p21 via the p21 -RE1-pGL3 enhancer by REST was evaluated using luciferase reporter gene assay as described previously [20] . DNA fragment of p21 gene with or without mutation or deletion of the p21-RE1 was PCR cloned into a PGL3 enhancer luciferase reporter vector (Supplementary Table 1 ). All constructs were confirmed by Sanger sequencing. 0.8 µg of each p21 -RE1-pGL3 enhancer construct was co-transfected with 0.2 µg of pRL-SV40 vector (Promega, E2231) into cultured P1 CMs in 96-well plates using Lipofectamine 3000 Reagents (Invitrogen). After 24 h transfection, cell lysates were processed for luciferase activity using the luciferase reporter system (Promega, E1980). Luciferase reporter activities were calculated as firefly luciferase normalized to Renilla luciferase luminescence. Biological triplicates were performed in technical triplicates for each vector. Immunostaining Immunostaining was performed on sections of paraffin-embedded embryos or hearts, as previously described [39] . Embryos or hearts were collected at the indicated stages and fixed in 4% PFA for 2 h, rinsed in PBS, dehydrated in 15 and 30% sucrose sequentially, embedded in optimal cutting temperature (OCT) compound and sectioned at 8-μm thickness. Heart sections were blocked with 5% horse serum for 1 h at room temperature before being incubated overnight at 4 temperature with the single or double staining with following antibodies diluted in blocking solution: TnT (Fisher Scientific, MS-295-P0, 1:400), PECAM1 (Santa, sc-1506, 1:400), REST (Antibodies-online, ABIN747683, 1:400 dilution), Ki67 (Abcam, ab66155, 1:200), P21 (Abcam, ab109199, 1:100 dilution), cleaved caspase-3 (CST, mAb #9664, 1:200), phosphorylated-histone3 (pH3) (Abcam, ab32107, 1:200), or aurora B (Abcam, ab2254,1:100). After three washes with PBS for 5 min each, samples were stained for 1 h at room temperature with fluorescent secondary antibodies followed by DAPI (4′,6-diamidino-2-phenylindole dihydrochloride) staining for nuclei visualization. Images were acquired and analyzed using a Zeiss fluorescence microscope with Axiovision image analysis software. For paraffin sections, 6-µm tissue sections were de-waxed in xylene, rehydrated in descending grades of alcohol and antigen-retried by incubating in sodium citrate for 10 min at 95 °C. After blocked with 5% horse serum for 60 min, sections were incubated with antibodies against NKX2.5 (Santa, sc-14033, 1:500) overnight at 4 °C, followed by incubation with biotinylated secondary antibodies (Vectastain, PK-6100) for 1 h and stained with DAB (Vector, SK-4100). Counterstaining with hematoxylin was used for visualization of nuclei. All immunostaining were performed on four sections per sample, and total four samples of each genotype and treatment group were experimented. 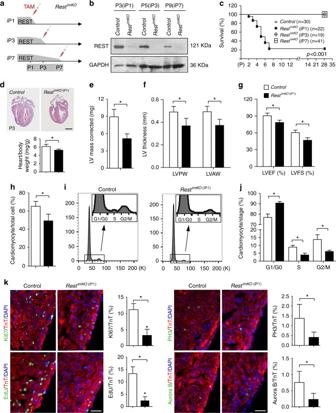Fig. 2 Restis required for neonatal cardiomyocyte proliferation and cardiac function.aA graph of experimental design for generating myocardialRestknockout (RestimKO) at different postnatal (P) stages using the inducibleTnTMerCreMerdeleter mice.bWestern blots showing effective deletion ofRest.cSurvival curve of control andRestimKOmice,p< 0.001, log-rank (Mantel–Cox) testing between mice withRestdeletion at different stages and control (Tam-treatedRest+/+;TnTMerCreMer/+mice).dRepresentative H&E staining and heart/body weight ratio revealing underdevelopedRestimKOhearts at P3 afterRestdeletion at P1.n= 5/group. Scale bar = 100 µm.e–gEchocardiography showing structure defects and decreased left ventricle function of P3RestimKO.n= 6 forRestimKO;n= 8 for Control.h–jFACS shows reduced percentage of cardiomyocytes isolated from P3RestimKOhearts (h) and arrested cell cycle of theRestimKOcardiomyocytes at G0/G1 phase (i,j).kImmunostaining for cell cycle markers indicating reduced proliferation ofRestnull cardiomyocytes.n= 4/group for FACS and immunostaining. Scale bar = 40 µm. Mean ± s.d., *p< 0.05, unpaired two-tailed Student’sttest Images were taken from six fields per section, processed using ImageJ software and counted blindly to genotype and treatment groups. EdU incorporation Proliferative cells were pulse labeled for 2 h by intraperitoneal injection of mice with 5-ethynyl-2′-deoxyuridine (EdU, 100 mg/kg). Hearts were then collected, fixed in 4% PFA, rinsed in PBS, soaked in 15 and 30% sucrose sequentially, embedded in OCT, and sectioned at 8-μm thickness. Sections were stained with antibodies against TnT (Fisher Scientific, MS-295-P0, 1:400) or REST (Antibodies-online, ABIN747683, 1:400), followed by EdU staining (Click-iT® EdU Alexa Fluor® 488 Imaging Kit, Life Technologies) and DAPI counterstaining (Vector lab, H1200). Stained sections were photographed under a Zeiss microscope, and images were processed for quantitative analysis as described above. Flow cytometry P3 ventricles of Rest knockout ( Rest imko ) mice and littermate controls of both sexes were digested into single cell suspension, fixed with 70% ethanol. CMs were stained with TnT antibodies (Fisher Scientific, MS-295-P0, 1:400) for 2 h at room temperature and then incubated with secondary antibodies (Alexa Fluor™ 488 Tyramide SuperBoost™ Kit, goat anti-mouse IgG). Cell pellets were re-suspended in FxCycle™ PI/RNase Staining Solution (Fisher Scientific, F10797) and analyzed on a FACStar Plus flow cytometer (Becton Dickinson, Franklin Lakes, NJ). An average of 10 4 CMs (FITC+) were collected in the gate from total cells per ventricle using forward and side scatter. We used pulse width versus pulse area as first gate on the single cell population and then applied this gate to the scatter plot to gate out cell debris. The combined gates were applied to the PI histogram plot to obtain the percentage of cells in each cell cycle phase. Apoptosis assay Apoptotic cells were visualized by TUNEL assay. Frozen sections were stained with TnT antibodies (Fisher Scientific, MS-295-P0, 1:400), followed by TUNEL staining using a DeadEndTM Fluorometric TUNEL kit (Promega). After DAPI counterstaining, sections were photographed under a Leica SP5 confocal microscope. Stained sections were photographed, and images were processed for quantitative analysis as described above. Statistics No statistical methods were used to predetermine sample size. Student’s t test (two-tailed) or one-way ANOVA analysis followed by Tukey’s, Sidak’s, or Bonferroni test was used for statistical difference between or among groups. The relationship between REST expression and cell proliferation during cardiac regeneration was analyzed by Pearson correlation coefficient. Survival rate of mice at various stages was calculated using log-rank (Mantel–Cox) test. Normality was assumed and variance was compared between or among groups. Sample size was determined based upon previous experience in the assessment of experimental variability. The investigators were not blinded to the group allocation during experiments and outcome assessment, unless stated otherwise. We chose the adequate statistic tests according to the data distribution to fulfill test assumptions. Statistical comparison for all quantitative assays was performed in at least three independent experiments. All numerical data were presented as mean ± s.d. and p value of <0.05 was considered as significant. Statistical analyses were performed using the SPSS v16.0 software (SPSS Inc., Chicago, IL). 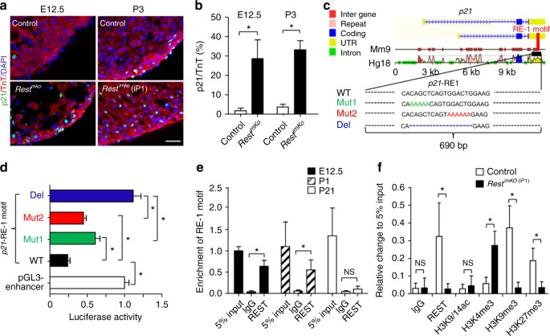Fig. 3 REST binds p21 to repress its expression.a,bImmunostaining (n= 4/group) showing upregulated p21 protein level in theRestdeleted E12.5 and P3 hearts. Scale bar = 40 µm.cTop, Sequence alignment ofp21between mouse and human indicating a conservedRE-1motif (red vertical line) located at the 3′ UTR. Bottom, Thep21-RE1 motif and its mutated (Mut) or deleted (Del) counterpart.dLuciferase reporter assays with a 690-bp mouse DNA fragment containing the wild type (WT), mutated, or deleted RE1 motif reveals that the intactp21-RE1 motif is required for repressing the reporter gene transcription in primary cultured P1 mouse cardiomyocytes.eqChIP using REST antibodies indicates enrichment ofp21-RE1 motif containing DNA fragments in the ventricles of E12.5 and P1, but not P21.fqChIP with P2 ventricles using the REST and histone mark antibodies showing the REST-dependent histone modification of thep21-RE1 motif.n= 3/group ford–f, mean ± s.d., *p< 0.05 by one-way ANOVA followed by Tukey’s test ind; unpaired Student’sttest inb,e,f. NS no significance Data availability Data supporting the findings of this study are available within the article and its Supplementary Information files. All relevant data are available from the authors on reasonable request. 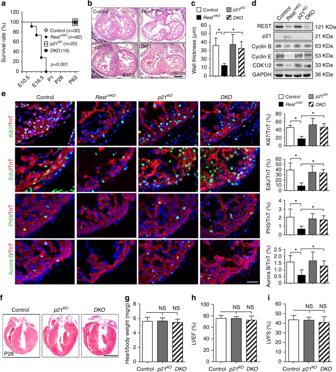Fig. 4 p21deletion rescues embryonic heart defects resulting from myocardialRestdeletion.aSurvival curve, no difference between control andp21null (p21KO) orp21/Restdouble knockout (DKO) group by log-rank (Mantel–Cox) test.p< 0.001 betweenRestmKOand each of other groups.b,cH&E-stained E12.5 heart sections showing that thin ventricular walls ofRestdeleted hearts are restored byp21deletion (n= 3/group). Scale bar = 100 μm.dRepresentative western blot revealing that upregulation of p21 and downregulation of Cyclin B, Cyclin E, and CDK1/2 in E12.5Restnull hearts are restored to the normal levels of control hearts byp21deletion.eImmunostaining for cell cycle markers indicating thatp21inactivation rescues the cell cycle defect resulting fromRestdeletion (n= 4/group). Scale bar = 40 μm.f–iH&E staining (fscale bar = 100 μm), ratio of heart/body weight (g), and echocardiography (h,i) showing that P28Rest/p21DKO mice have cardiac structure and function comparable to control littermates (n= 6–8/group). Mean ± s.d. *p< 0.05 by one-way ANOVA followed by Tukey’s test. NS no significance 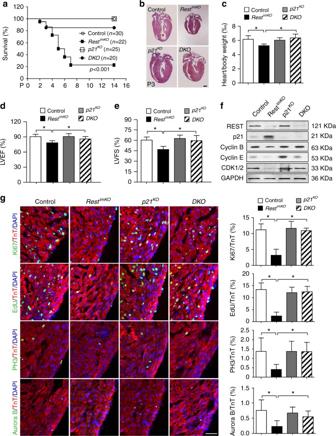Fig. 5 p21deletion rescues neonatal heart defects resulting fromRestdeletion.aSurvival curve, no difference between control andp21null (p21KO) orp21/Restdouble knockout (DKO) group by log-rank (Mantel–Cox) test.p< 0.001 betweenRestimKOand each of other groups.b,cH&E-stained P3 heart sections showing that underdevelopedRestnull hearts are restored byp21deletion (n= 5/group). Scale bar = 100 μm.d,eEchocardiograph showingp21knockout rescues cardiac function resulting fromRestdeletion at P1 (n= 6–8/group).fRepresentative western blot revealing upregulation of p21 and downregulation of Cyclin B, Cyclin E, and CDK1/2 in P3Restnull hearts are restored byp21deletion to the normal levels of control hearts.gImmunostaining for cell cycle markers indicatingp21inactivation rescues the cell cycle defect resulting fromRestdeletion (n= 4/group). Scale bar = 40 μm. Controls were the Tam-treatedRest+/+;TnTMerCreMer/+mice. Mean ± s.d. *p< 0.05 by one-way ANOVA followed by Tukey’s test 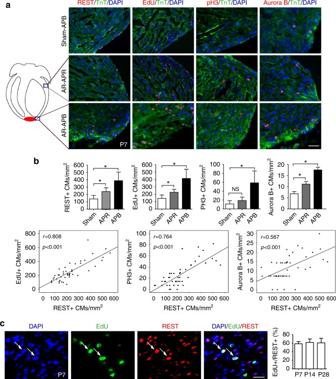Fig. 6 Co-upregulation of REST and cardiomyocyte proliferation in injured neonatal hearts.a,bQuantitative immunofluorescence (aScale bar = 40 μm.) and scatter plotbshowing increased expression of REST and its positive relation with the expression of cell cycle markers in cardiomyocytes. Average counts from six fields/section, four sections/ventricle, four ventricles/stage at P7, P14, and P28, mean ± s.d. *p< 0.05 by one-way ANOVA followed by Tukey’s test. APB/APR apex border/apex remote.cCo-immunofluorescence showing consistently ~60% of EdU+ cells express REST (arrow) in regenerating neonatal hearts. Scale bar = 10 μm. Data are presented as mean ± s.d. (n= 4/stage) 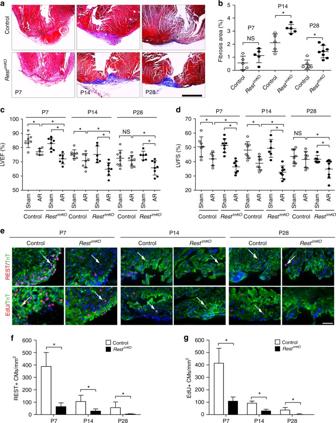Fig. 7 Restis required for regeneration of injured neonatal hearts.a,bQuantitative Masson’s trichrome staining shows increased cardiac fibrosis in mice with induced myocardialRestdeletion at P3 and injured by apex ablation at P4,n= 5–8/group. Scale bar = 100 μm.c,dEchocardiography indicating reduced cardiac function of myocardialRestnull mice after injury,n= 6–8/group.e–gQuantitative immunofluorescence (n= 4/group) showing decreased EdU+ cardiomyocytes in regenerating hearts in mice withRestdeletion. Scale bar = 40 μm. Mean ± s.d.p< 0.05 by two-way ANOVA followed by Sidak’s test inb–d; unpaired two-tailed Student’sttest inf,g 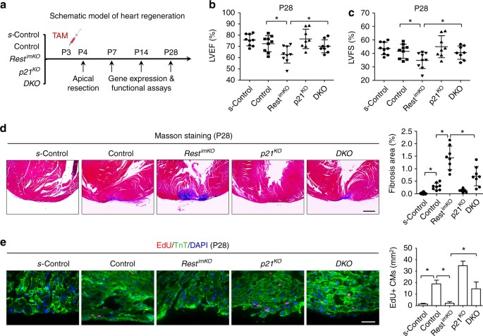Fig. 8 REST-dependentp21expression is required for cardiac regeneration.aSchematic diagram showing experimental procedure of cardiac apex resection (AR) on neonatal mice.b,cEchocardiography indicates that mice with control (n= 9), singlep21knockout (p21KO,n= 8), and double knockout ofRestandp21(DKO,n= 8) injured hearts have cardiac function comparable to that of the sham-operated control (s-Control,n= 9) at P28. InjuredRestsingle knockout (RestimKO,n= 9) hearts have significantly decreased left ventricular function comparable to injured control.d,eQuantitative Masson’s trichrome staining (n= 8/group) (dScale bar = 100 µm) and EdU assays (n= 4/group) (eScale bar = 40 µm) showingp21inactivation reduces the cardiac fibrosis and rescues cardiomyocyte proliferation defect in the injured apex resulting fromRestdeletion. Mean ± s.d. *p< 0.05 by one-way ANOVA followed by Bonferroni test. NS no significance The RNA-Seq data have been downloaded from the NIH GEO database with accession code GSE80378.